Exceptional mobility of an advancing rhyolitic obsidian flow at Cordón Caulle volcano in Chile The emplacement mechanisms of rhyolitic lava flows are enigmatic and, despite high lava viscosities and low inferred effusion rates, can result in remarkably, laterally extensive (>30 km) flow fields. Here we present the first observations of an active, extensive rhyolitic lava flow field from the 2011–2012 eruption at Cordón Caulle, Chile. We combine high-resolution four-dimensional flow front models, created using automated photo reconstruction techniques, with sequential satellite imagery. Late-stage evolution greatly extended the compound lava flow field, with localized extrusion from stalled, ~35 m-thick flow margins creating >80 breakout lobes. In January 2013, flow front advance continued ~3.6 km from the vent, despite detectable lava supply ceasing 6–8 months earlier. This illustrates how efficient thermal insulation by the lava carapace promotes prolonged within-flow horizontal lava transport, boosting the extent of the flow. The unexpected similarities with compound basaltic lava flow fields point towards a unifying model of lava emplacement. Controls on lava flow lengths and advance rates include lava viscosity and yield strength, together with effusion rate and topography [1] , [2] , [3] . As lava viscosity and yield strength increase with melt silica content [4] , high-silica lavas are generally considerably thicker, shorter and more slow-moving than basaltic lavas [2] , [3] , [5] , [6] , although crystal-poor rhyolitic lava may be significantly less viscous than crystal-rich andesite or dacite. Formation of an insulating crust reduces heat loss and significantly enhances lava mobility [2] , [3] . Crust formation is known to be important in basaltic lavas [7] , and extensive tube-fed lavas are commonly compound (consisting of multiple flow units [8] , [9] ). Basaltic flow fields often advance through extrusion from stalled flow fronts [8] , [10] . Despite their high viscosity and inferred effusion rates of <100 m 3 s −1 , some rhyolitic lavas can flow for distances exceeding 30 km (ref. 11 ) and produce flows with volumes of up to 10–20 km 3 (refs 12 , 13 ). Ogives indicate folding of ~10 m-thick surface crusts [5] , which may boost flow mobility by providing effective thermal insulation [13] . However, unlike basaltic flow models, existing models of rhyolitic flow emplacement focus on the inflation of single lava flow units once flow fronts have stalled [14] , [15] , [16] . Before the 2011–2012 eruption of Cordón Caulle, the 2008–2009 eruption at Chaitén had provided the only opportunity to observe the emplacement of rhyolitic lava, with both exogenous and endogenous growth of a complex of domes and spines between May 2008 and late 2009 (refs 17 , 18 ). The mean effusion rate of the crystal-poor, high-silica rhyolite (75 wt% SiO 2 ) was 66 m 3 s −1 over the first 2 weeks and the total erupted lava volume was ~0.8 km 3 . Notably, no extensive rhyolitic flow was generated, with lava extending <1 km from the vent [18] . Constraints on the evolution of extensive rhyolite lava flows have been previously derived indirectly from analogue experiments [2] , viscous flow models [5] , [19] and thermal models [13] . In contrast, the temporal evolution of frequently observed basaltic lava flow fields is well constrained [7] , [10] , [20] , and transitions from simple to compound flow fields that consist of multiple flow units are well documented [8] , [9] . In compound basaltic flows, cessation of flow front advance triggers channel overflows and breaches, or flow inflation and lava extrusion at flow fronts via localized breakouts or squeeze-ups [10] . Long-term processes in compound basaltic lava flow fields are therefore both vertical (flow inflation and tumulus formation) and horizontal (creation of breakouts). Some cross-compositional commonality in lava effusion and emplacement mechanisms has been identified, including localized lava extrusion at dacitic lava flow margins [21] that has a direct basaltic equivalent [10] , [22] . However, similarities between rhyolitic and basaltic emplacement are largely unquantified, and advance processes in rhyolitic lava flow fields are poorly understood. Our study addresses this issue by applying quantitative three-dimensional (3D) imaging techniques [23] to the first extensive rhyolitic lava flow field to be observed in evolution, emplaced during the 2011–2012 eruption of Cordón Caulle, Chile. Puyehue–Cordón Caulle (40.5 °S) is a large basaltic-to-rhyolitic volcanic complex within the Andean Southern volcanic zone, 125 km northeast of Puerto Montt, Chile ( Fig. 1 ). The 20-km-long, NW-trending Cordón Caulle fissure complex ( Fig. 1 ) has produced ~9 km 3 of rhyodacitic to rhyolitic lavas and pyroclastic deposits since 16.5 ka [24] . Cordón Caulle has produced two major historic eruptions, in 1921–1922; and 1960, in which 0.25–0.3 km 3 of rhyolitic magma (dense rock equivalent; 69.5–70.3 wt % SiO 2 ) was erupted from ≤5.5 km-long fissures [25] . 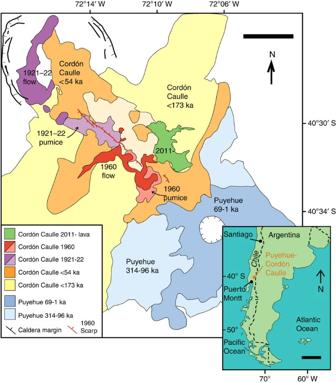Figure 1: The Puyehue–Cordón Caulle volcanic complex. Highly simplified geological map of the Puyehue–Cordón Caulle volcanic complex, redrawn from Singeret al.24and Laraet al.25The Cordón Caulle volcanic system forms a 20-km-long and 4-km-wide ridge oriented NW-SE. The main fault scarps associated with the 1960 eruption25are shown. Scale bar, 5 km in length. Inset: map indicating position of Cordón Caulle volcanic complex in southern Chile, redrawn from ref.30. Scale bar, 100 km in length. Figure 1: The Puyehue–Cordón Caulle volcanic complex. Highly simplified geological map of the Puyehue–Cordón Caulle volcanic complex, redrawn from Singer et al. [24] and Lara et al. [25] The Cordón Caulle volcanic system forms a 20-km-long and 4-km-wide ridge oriented NW-SE. The main fault scarps associated with the 1960 eruption [25] are shown. Scale bar, 5 km in length. Inset: map indicating position of Cordón Caulle volcanic complex in southern Chile, redrawn from ref. 30 . Scale bar, 100 km in length. Full size image An explosive eruption (0.2–0.4 km 3 dense rock equivalent pyroclastic deposits) commenced on 4 June 2011, with a 27-h-long initial Plinian phase (≤15 km plume height) [26] , [27] . Ash plume heights had decreased to 2–5 km by January 2012, when our observations were collected, and ash emissions ended in June 2012. A 50-m-wide, 150-m-long lava flow was first observed on 20 June 2011 (ref. 28 ). Although lava outflow at the vent arguably ended on 15 March 2012, when tremors ceased [29] , the flow field continued to evolve into January 2013, when we witnessed rockfall at an advancing breakout. Lava flow field evolution was captured [30] by the Earth Observing-1 spacecraft ( Fig. 2 ). The initial lava discharge rate was estimated [31] to be 20–60 m 3 s −1 and the discharged lava volume was ~0.4 km 3 by April 2012 (C. Silva Parejas, personal communication). Lava whole-rock composition is rhyolitic [26] , with 69.8–70.1 wt% SiO 2 and 7.8 wt% Na 2 O+K 2 O, and glass water contents are <0.2 wt% (J.M. Castro, manuscript in preparation). 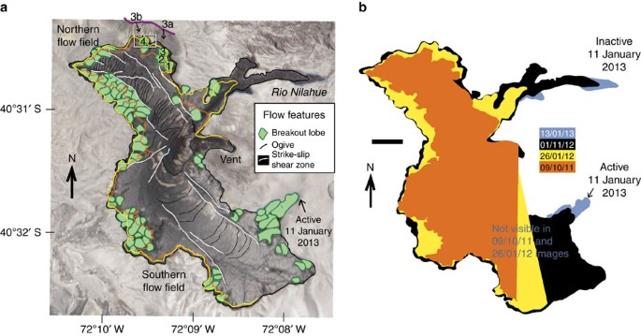Figure 2: Overview of lava flow field evolution. (a) Advanced Land Imager image from 13 January 2013, showing the rhyolitic flow field, with evolving marginal position indicated by a series of flow lines: 9 October 2011 (orange), 26 January 2012 (yellow), 1 November (black) and 13 January 2013 (blue). Over 80 breakout lobes are labelled; these exclusively occur outside marginal shear zones and the overwhelming majority formed after 9 October 2011. Numbered breakout lobes (1–4) correspond with lobes shown inFig. 3. The bold purple line at the top of the figure indicates the traverse followed during imaging of the flow front, and labels 3a and 3b indicate locations of images inFig. 3a and b, respectively; the white box indicates the location ofFig. 4a. Scale bar, 500 m in length. (b) Four snapshots of the advancing flow margin between 9 October 2011 and 13 January 2013 from satellite imagery. The principal change between 9 October 2011 and 26 January 2012 was flow widening of up to ~400 m via breakout lobe formation. Post-26 January 2012 evolution was dominated by >1 km advance of the eastern flow and post-1 November 2012 evolution restricted to advance (<500 m) of the eastern flow and southeastern breakout lobes. Scale bar, 500 m in length. Figure 2: Overview of lava flow field evolution. ( a ) Advanced Land Imager image from 13 January 2013, showing the rhyolitic flow field, with evolving marginal position indicated by a series of flow lines: 9 October 2011 (orange), 26 January 2012 (yellow), 1 November (black) and 13 January 2013 (blue). Over 80 breakout lobes are labelled; these exclusively occur outside marginal shear zones and the overwhelming majority formed after 9 October 2011. Numbered breakout lobes (1–4) correspond with lobes shown in Fig. 3 . The bold purple line at the top of the figure indicates the traverse followed during imaging of the flow front, and labels 3a and 3b indicate locations of images in Fig. 3a and b , respectively; the white box indicates the location of Fig. 4a . Scale bar, 500 m in length. ( b ) Four snapshots of the advancing flow margin between 9 October 2011 and 13 January 2013 from satellite imagery. The principal change between 9 October 2011 and 26 January 2012 was flow widening of up to ~400 m via breakout lobe formation. Post-26 January 2012 evolution was dominated by >1 km advance of the eastern flow and post-1 November 2012 evolution restricted to advance (<500 m) of the eastern flow and southeastern breakout lobes. Scale bar, 500 m in length. Full size image Here we show that localized extrusion from the margins of the rhyolitic lava flow field at Cordón Caulle greatly extended the flow field during 18 months of flow evolution, and that this process continued for several months after the supply of lava at the vent ceased. Our results demonstrate how efficient thermal insulation by the lava crust allows prolonged advance of compound rhyolitic flow fields, and reveal unexpected commonality with processes at basaltic lava flow fields. Ground-based imaging of the evolving lava flow field Imaging of the northern lava flow field was conducted on 3–4 and 10 January 2012. In 2012, vent activity was characterized by semicontinuous ash jetting punctuated by Vulcanian-like blasts, creating a 2-km-high ash plume [32] . Visual observations and digital photographs for 3D reconstruction were collected during ~1-km-long traverses of a ridge directly overlooking the northern flow margin ( Fig. 2a ). See Methods for details of the automated photo reconstruction techniques employed. We noted structural and textural features typical of documented obsidian flows in the lava, such as ogives on the flow surface [5] , [6] , [16] , [19] and zones of variably vesicular glassy lava [14] , [15] , [16] , including coarsely vesicular pumice. On 4 January 2012, the lava flow front was characterized by two dominant facies ( Fig. 3 ). Predominant rubbly lava was ~30–40 m thick and mantled by unstable talus. Angular, rotated lava blocks ranged from tens of centimetres to several metres across. Larger dissected blocks displayed red, oxidized interiors, with pale upper surfaces due to vapour-phase precipitates and ash cover. Intact lava locally protruded through the talus-covered upper carapace ( Fig. 3b ). A near-linear, 10–30 m-high scarp bounding the rubbly lava facies ( Fig. 3a ) corresponded to a channel-bounding shear zone evident in satellite images ( Fig. 2a ). 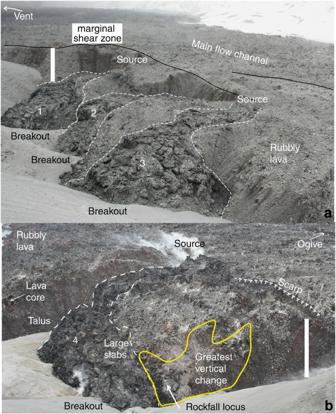Figure 3: Images of breakouts at lava margin. (a) View of northeastern lava flow margin, looking south, on 4 January 2012. Three prominent lava breakouts (1–3) are characterized by darker colouring, surface of large lava slabs up to 10 m in length and their thinness relative to the main body of the lava flow. Breakout source regions correspond with a marginal shear zone. Scale bar, 30 m in length. (b) Overview of the breakout imaged inFig. 4a, looking southeast on 10 January 2012. The flow-folded lava slabs and embryonic talus slope of the breakout contrasts with rubbly lava to the left. The zone of greatest vertical change between 4 and 10 January 2012 is indicated (yellow line). Note the strong localized degassing occurring at the breakout source. Scale bar, 30 m in length. Figure 3: Images of breakouts at lava margin. ( a ) View of northeastern lava flow margin, looking south, on 4 January 2012. Three prominent lava breakouts (1–3) are characterized by darker colouring, surface of large lava slabs up to 10 m in length and their thinness relative to the main body of the lava flow. Breakout source regions correspond with a marginal shear zone. Scale bar, 30 m in length. ( b ) Overview of the breakout imaged in Fig. 4a , looking southeast on 10 January 2012. The flow-folded lava slabs and embryonic talus slope of the breakout contrasts with rubbly lava to the left. The zone of greatest vertical change between 4 and 10 January 2012 is indicated (yellow line). Note the strong localized degassing occurring at the breakout source. Scale bar, 30 m in length. Full size image Lobes of darker, slabby lava 50–100 m across and ~20 m thick protruded from the flow margin, forming largely talus-free lava bodies extending roughly perpendicular to the channel margin and overlying the talus apron of the rubbly lava. We term these breakout lobes. Their upper surfaces consisted of smooth, locally folded dark gray lava slabs mostly 5–15 m across but occasionally significantly larger ( Fig. 3b ), with many cut by crevasse-like crease structures and en-echelon tensional fractures. During ~2 h of observation, the toe of the breakout lobe was the most frequent location of small-volume (~1–3 m 3 ) rockfalls ( Supplementary Movie 1 ), which occurred at ~1–10 min intervals and also originated from core material in the rubbly lava ( Supplementary Movie 2 ). Two 3D point clouds were generated and interpolated into digital elevation models for 4 and 10 January 2012 to yield surface change over this period ( Fig. 4a ). Vertical and horizontal movement was spatially heterogeneous, indicating localized advance, inflation and collapse of lava. The rubbly lava experienced relatively uniform vertical inflation (~0.5–3 m), with greater vertical change locally associated with exposed core lava in the upper talus slope ( Fig. 4b ). Horizontal displacements indicate general northeast movement of <10 m, consistent with the overall spreading direction of lava perpendicular to the nearest channel margin ( Fig. 2a ). 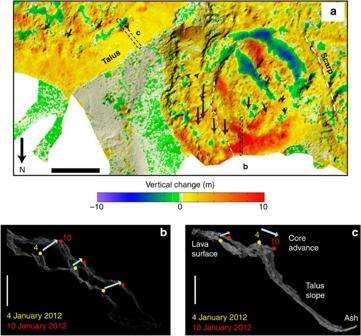Figure 4: Evolving breakout morphology 4–10 January 2012. (a) Map of vertical change over 4–10 January at the lava flow margin. White represents no data and areas with <0.2 m vertical change are transparent, revealing gray-shaded topography in areas of minimal variation. The lava shows overall inflation, with some areas of apparent decrease most probably resulting from horizontal movement of the undulose surface. Horizontal displacements of individually identifiable features are indicated by the arrow trunk lengths, with the greatest velocities associated with the slabby area of the breakout region. The greatest vertical changes, directly to the west of the breakout margin, reflect combined advance and inflation of the flow front. Dashed boxes b and c indicate the location of cross-sections in panelsbandc. Scale bar, 50 m in length. (b) Cross-section through the original point cloud data in the zone of greatest vertical change, showing the trajectory (arrows) of labelled topographic features. Scale bar, 10 m in length. (c) Cross-section through the margin of the rubbly lava, showing greatest change of the lava core, which has both advanced and moved downwards. The lava surface (left) has undergone modest advance and little inflation, whereas there is little change in the talus slope. Scale bar, 10 m in length. Figure 4: Evolving breakout morphology 4–10 January 2012. ( a ) Map of vertical change over 4–10 January at the lava flow margin. White represents no data and areas with <0.2 m vertical change are transparent, revealing gray-shaded topography in areas of minimal variation. The lava shows overall inflation, with some areas of apparent decrease most probably resulting from horizontal movement of the undulose surface. Horizontal displacements of individually identifiable features are indicated by the arrow trunk lengths, with the greatest velocities associated with the slabby area of the breakout region. The greatest vertical changes, directly to the west of the breakout margin, reflect combined advance and inflation of the flow front. Dashed boxes b and c indicate the location of cross-sections in panels b and c . Scale bar, 50 m in length. ( b ) Cross-section through the original point cloud data in the zone of greatest vertical change, showing the trajectory (arrows) of labelled topographic features. Scale bar, 10 m in length. ( c ) Cross-section through the margin of the rubbly lava, showing greatest change of the lava core, which has both advanced and moved downwards. The lava surface (left) has undergone modest advance and little inflation, whereas there is little change in the talus slope. Scale bar, 10 m in length. Full size image The breakout lobe underwent more heterogeneous vertical inflation ( Fig. 4a ), with strongest vertical change (4–11 m) in zones of slab rotation, break-up and most frequent rockfall events at the lobe margin. Horizontal displacements were significantly greater than that in the rubbly lava, with northward movement of ~20 m in the central part of the lobe. Between 4 and 10 January, the propagation and coalescence of tensile fractures in large lava slabs ( Fig. 5 ) led to their break-up into smaller blocks to create an incipient talus mantle. 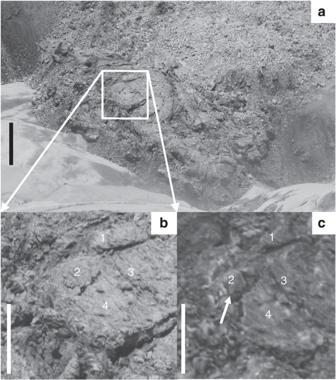Figure 5: Progressive fracturing in evolving breakout lobe. (a) Overview of breakout lobe 4 on 4 January, with white box indicating the location ofb. Breakout location indicated inFig. 2aand scale bar, 10 m in length. (b) Close-up of this 4 January image, showing large lava slabs cut by incipient tension fractures metres in length. The crack between 2 and 3 is <0.5 m wide and cuts an otherwise mostly intact slab. Scale bar, 5 m in length. (c) Close-up of the same area asbon 10 January 2012, with the corresponding locations marked by the same numbers as inb. The darker colour is due to rainfall having washed ash from the lava surface. The incipient crack between 2 and 3 has now widened and branched (white arrow), leading to the break-up of an ~5-m-wide portion of the slab to smaller blocks 0.3–2 m across. Through this process, breakouts mature through slab break-up, eventually creating more rubbly material indistinguishable from the rubbly flow facies (Fig. 6). Scale bar, 5 m in length. Figure 5: Progressive fracturing in evolving breakout lobe. ( a ) Overview of breakout lobe 4 on 4 January, with white box indicating the location of b . Breakout location indicated in Fig. 2a and scale bar, 10 m in length. ( b ) Close-up of this 4 January image, showing large lava slabs cut by incipient tension fractures metres in length. The crack between 2 and 3 is <0.5 m wide and cuts an otherwise mostly intact slab. Scale bar, 5 m in length. ( c ) Close-up of the same area as b on 10 January 2012, with the corresponding locations marked by the same numbers as in b . The darker colour is due to rainfall having washed ash from the lava surface. The incipient crack between 2 and 3 has now widened and branched (white arrow), leading to the break-up of an ~5-m-wide portion of the slab to smaller blocks 0.3–2 m across. Through this process, breakouts mature through slab break-up, eventually creating more rubbly material indistinguishable from the rubbly flow facies ( Fig. 6 ). Scale bar, 5 m in length. Full size image Broad-scale lava flow field evolution Sequential satellite images of the evolving lava flow field ( Fig. 2 ) indicate increasing flow complexity, with flow front breakouts first appearing between 18 August and 9 October 2011, 64–116 days after the lava-producing phase began, and dominating lava evolution from October 2011 ( Fig. 2 ). These breakouts followed the initial main channel flow (June–August 2011). This change reflects how progressive stagnation of the flow fronts and sides, probably because of topographic constraints and cooling-driven crustal thickening [9] , drove the transition from a simple to a compound lava flow field. The development of strike-slip marginal shear zones allowed stalling of channel margins despite continued lava advance at channel centres ( Fig. 6 ). The change in the mode of flow emplacement also mirrors the transitions from axisymmetric to more complex lobate, platy and spiny morphologies observed in analogue experiments [2] with dwindling effusion rate. The northern flow field width increased by ~100–400 m between 9 October 2011 and 26 January 2012 at ~1–4 m per day, predominantly because of breakout extrusion from both margins. This rate broadly matches our surface velocity measurements from one margin (1.5–3 m per day), indicating that the advance rates observed in the field are representative of the broader flow field evolution. 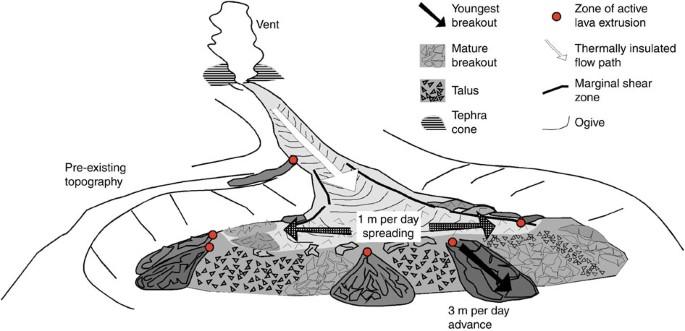Figure 6: Schematic lava emplacement model. Cartoon indicating the mode of compound lava field evolution between October 2011 and January 2012, illustrating the localized nature of breakout extrusion at lava margins and various stages in the evolution of breakouts from slabby to rubbly lava. Much of the lava margin comprises a collage of lava breakouts of different ages and varying maturity. Figure 6: Schematic lava emplacement model. Cartoon indicating the mode of compound lava field evolution between October 2011 and January 2012, illustrating the localized nature of breakout extrusion at lava margins and various stages in the evolution of breakouts from slabby to rubbly lava. Much of the lava margin comprises a collage of lava breakouts of different ages and varying maturity. Full size image The >80 breakout lobes visible in the 13 January 2013 image ( Fig. 2a ) display a narrow range of lengths (mostly ~50–100 m). However, one breakout formed a far longer, rapidly advancing new lava channel to the east ( Fig. 2 ) because of overtopping a topographic barrier and flow down a steepening slope. Elsewhere, breakouts have limited volumes and lifespans, and earlier breakout lobes are either engulfed by the main flow field or overridden by later breakouts ( Fig. 6 ). Lava emission from breakouts >3 km from the lava source vent highlight the effective thermal insulation of the flow carapace [13] , lending remarkable mobility to highly viscous lava, which does not require, but may be enhanced by, downward-sloping underlying topography. Indeed, significant flow field evolution continued after November 2012, and we directly observed advance of southeastern breakout lava on 11 January 2013, 8 months after the lava supply at the vent halted ( Supplementary Movies 1 and 4 ). We estimate the lava path length from the vent to this breakout to be 3.6±0.3 km ( Fig. 2a ). If heat production within the flow is neglected, cooling front propagation into the lava can be roughly approximated [33] as 2.3( kt ) 0.5 , where k is thermal diffusivity and t is the time in seconds. Using a value [34] of thermal diffusivity for rhyolite of 5.5 × 10 −7 m 2 s −1 , a 35-m-thick lava would take over 3 years to solidify, leaving considerable time for the supply of lava to its margins, allowing continued flow advance, after the eruption ceased. In reality, heat production by shear heating [35] at marginal shear zones and/or spherulite crystallization in the flow interior [36] may serve to buffer cooling and prolong lava advance. Rhyolitic breakouts share many features with breakouts and squeeze-ups documented in stalling and compound basaltic flow fields [10] , [22] . With both compositions, lava breaks out from stalled lava flow fronts and channel margins where shear stresses are highest. Surface textures are slabby, indicating ductile extrusion on shear surfaces that extend back into the lava interior, and slab sizes far exceed block sizes in neighbouring 'a'a/rubbly lava [10] . Brittle deformation becomes increasingly important as slabs cool, with inflation triggering slab fracturing and evolution towards rubbly flow facies ( Figs 5 and 6 ). We noted significant evolution of breakout lava over a 6-day period, with break-up of initially coherent lava slabs, inflation, steepening and the onset of talus formation, as breakout lava was maturing into the predominantly thicker, rubbly lava ( Figs 5 and 6 ). Reducing slab size may therefore be a proxy for lava maturity rather than necessarily indicating lower effusion rates [37] . During the observation period, breakout horizontal velocities far exceeded vertical velocities ( Fig. 4 ) reflecting primarily horizontal flow rather than endogenous inflation. In this respect, the endogenous growth more closely matches that of basaltic lava flows [10] rather than previous interpretations and observations of high-silica rhyolites [6] , [16] , [17] , [18] . Breakouts created an embayed lava margin that appears typical of many low-silica rhyolite flows (for example, Laugahraun in Iceland), indicating that compound rhyolitic lavas may be commonplace, although hitherto unrecognized. Shear zones at the margins of the main channel are sites of localized ductile shear and loci for lava breakouts. Repeated extrusion of breakout lobes from lava margins may therefore create complex, superimposed internal structures related to strain localization and lateral flow, consistent with field observations of dissected small-volume, topographically confined rhyolitic lava bodies [38] . Our observations highlight the thermal efficiency of rhyolitic flows, which greatly increases their mobility and lengthens their timescale of potentially hazardous advance. Endogenic flow inflation, flow front advance by breakouts from insulated flow cores and transitions from juvenile slabby to mature rubbly flow textures are all processes observed syn-eruptively for the first time in a rhyolitic lava flow. These processes have previously been documented from basaltic flows, and thus point towards universal models of compound flow development that transcend orders of magnitude differences in magma rheology. Further studies of the Cordón Caulle lava will provide new insights into additional poorly constrained aspects of obsidian flow emplacement, which include viscous and yield strength controls on flow advance and the timescales of crust formation and deformation, plus lava devitrification and cooling. Terrestrial 3D imaging techniques Photogrammetry and other terrestrial imaging techniques are powerful tools for tracking the morphological evolution of lavas and domes [39] , [40] , [41] , and can be used in concert with satellite remote sensing techniques [42] . More recently, construction of 3D models using structure-from-motion (SfM) and multiview-stereo computer vision techniques allows quantitative interpretation of the temporal evolution of lava flow fields and silicic domes [43] , [44] , [45] . Here we employ these techniques to follow rhyolitic lava flow evolution at Cordón Caulle. A total of 1,258 images were collected in two surveys (4 and 10 January 2012) using a Canon 450D digital SLR camera with a 28-mm lens. Between two and eight images of the lava flow field were collected approximately every 15 m over a ~1-km-long traverse parallel to the flow margin ( Fig. 2a ). During the traverse of 10 January, image acquisition was accompanied by simultaneous logging of the photographer position using a handheld global positioning system (GPS) device. Each image set was processed into 3D point clouds in arbitrary coordinate systems by a freely available SfM and multiview-stereo workflow package ( http://www.blog.neonascent.net/archives/bundler-photogrammetry-package/ by J. Harle) [23] . To scale and geo-reference the point clouds, real-world camera locations were estimated for the 10 January survey by interpolating position from the GPS data for the time of each image acquisition. The best transform (a scaling, rotation and translation) to convert the camera positions determined in the SfM coordinate system to the real-world estimates was then calculated using sfm_georef (v2.3) software [23] , and the results were used to transform the point cloud. The root mean squared error between the GPS-estimated camera positions and those in the transformed model was 4.6 m, and was probably dominated by error in the GPS coordinates. To geo-reference the 4 January survey (for which GPS data were not available), static features were identified in both image sets and their real-world coordinates derived from the geo-referenced 10 January survey. These features were then used as control points to determine the geo-referencing transform for the survey of 4 January. The resulting root mean squared error between the control point coordinates in the 10 January and the transformed 4 January survey is 0.2 m, giving an indication of the quality of the relative registration between the two surveys. To derive the digital elevation models, regions of the 3D point clouds (as shown by the extent given in Fig. 4 ) were interpolated using Surfer software ( http://www.goldensoftware.com/products/surfer ). To determine 3D displacement vectors ( Fig. 4a ), sfm_georef was used to obtain the 3D coordinates of surface features that could be observed in both image sets (for example, the tops of distinctive blocks). Sfm_georef is available at http://www.lancs.ac.uk/staff/jamesm/software/sfm_georef.htm . How to cite this article: Tuffen, H. et al. Exceptional mobility of an advancing rhyolitic obsidian flow at Cordón Caulle volcano in Chile. Nat. Commun. 4:2709 doi: 10.1038/ncomms3709 (2013).